Photoconductive response in organic charge transfer interfaces with high quantum efficiency Organic semiconductors have unique optical, mechanical and electronic properties that can be combined with customized chemical functionality. In the crystalline form, determinant features for electronic applications, such as molecular purity, the charge mobility or the exciton diffusion length, reveal a superior improved performance when compared with materials in a more disordered form. However, the use of organic single crystals in devices is still limited to a few applications, such as field-effect transistors. Here we report the first example of photoconductive behaviour of single-crystal charge-transfer interfaces. The system composed of rubrene and 7,7,8,8-tetracyanoquinodimethane presents a responsivity reaching 1 A W −1 , corresponding to an external quantum efficiency of nearly 100%. This result opens the possibility of using organic single-crystal interfaces in photonic applications. Charge transfer through organic interfaces is an essential process for optoelectronic devices, such as organic photovoltaics, photodetectors and light-emitting diodes [1] , [2] . Indeed, the use of a donor–acceptor interface has boosted the efficiency of organic solar cells and remains one of the benchmarks of the field [3] , [4] . Excitons formed in the semiconductor layer are effectively separated at the donor–acceptor junction, leading to reported organic solar cell efficiencies in the 6–8% range [5] . Efforts to keep improving performance have been limited by factors related to optical absorption, exciton dynamics, charge-carrier mobility and its collection at the electrodes. Among the most relevant parameters to the performance of excitonic devices is the exciton diffusion length, L EX , usually much smaller, 10–50 nm, than the optical absorption length, 1/α, typically ~1 μm in organic semiconductors [6] . This leads to active layers of opposite ideal depth; thick layers for maximum light absorption and thin layers for an efficient exciton diffusion reaching the donor–acceptor heterojunction. Strategies to maximize efficiency have been envisioned, such as thin planar multilayers [7] , or blends [8] , [9] of polycrystalline or amorphous films, all aiming to combine the enlargement of the donor–acceptor contact area and the reduction of the exciton path. Unfortunately, limitations arouse because of disorder effects, morphology constrains and charge trapping associated with different trap energies and densities on uncontrolled grain boundaries [4] , [6] . For example, in polymer–fullerene bulk heterojunctions, there is a relatively unfavourable intermixing of the two components, resulting in a dispersion of the acceptor on the polymer matrix, limiting the drift length, and similarly the electrical fill factor, due to the recombination of holes with electrons trapped on isolated clusters [10] , [11] . In organic photodetectors, such charge trapping has been used to enhance photoconductivity gain, but at the expense of a high operating voltage [12] or incorporating rare and toxic inorganic materials in the composite matrix [13] , which limit the applications of these systems. In single-crystal organic semiconductors, the disorder effect is negligible and the highly organized molecular lattices promote orbital overlap, improving charge transport. This is clearly observed in single-crystal field-effect transistors, where both electron and hole mobilities are higher (1–10 cm 2 V −1 s −1 ) than what it is typically observed in devices based on polycrystalline or amorphous films (10 −3 cm 2 V −1 s −1 ) (refs 14 , 15 , 16 ). The surface modification using self-assembled monolayer (SAM) can also lead to high carrier density [17] . Moreover, crystallinity and, particularly trap-free single crystals, can lead to long-range exciton diffusion due to very efficient singlet–triplet exciton relaxation. Exciton diffusion over microscopic distances (2–8 μm) has recently been observed in rubrene single crystals due to singlet fission and subsequent migration of the long-lived triplet exciton to the crystal surface, where it then splits into free carriers [18] . In that work, the use of a top layer of an exciton splitter leads to a significant increase in the photoconductivity of rubrene. The advantages of using crystalline compounds over alloys or amorphous materials are well known among inorganic photovoltaic. An illustrative example can be found in silicon (Si), where the disordered distribution of hydrogen bond length and bond angles in amorphous Si disturbs the long-range order of the crystalline silicon lattice order, changing the optical and electronic properties and creating deep traps, which consequently lead to a cell efficiency less than half of crystalline Si solar cells cells [19] , [20] . Here we show that high photoconductivity gain can be obtained in a donor–acceptor system composed of highly ordered molecular crystals of two different organic compounds: rubrene and 7,7,8,8-tetracyanoquinodimethane (TCNQ). Both materials are large-gap organic semiconductors (more than 2 eV), forming molecular stacks in their crystalline structure ( Fig. 1 ) and having a high carrier mobility (hole mobility of 20 cm 2 V −1 s −1 in rubrene and electron mobility of 0.5 cm 2 V −1 s −1 in TCNQ, as measured in field-effect transistors [15] , [21] , [22] ). As a consequence of the large highest occupied molecular orbital–lowest unoccupied molecular orbital (HOMO–LUMO) gap, the conductivity of the two materials in the pure form is extremely small, as well as the quantum efficiency (max. ~10 −4 ) for photogeneration of carriers in single crystals and thin films [23] , [24] . The combination of two single crystals of a donor and acceptor materials forms a p–n heterojunction, in an analogue structure commonly used in inorganic semiconductors, in devices such as photodiodes or photodetectors. Such devices, based on crystalline organic semiconductors, have not previously been accomplished. 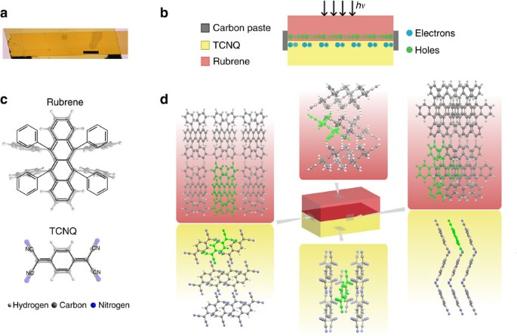Figure 1: Rubrene–TCNQ molecular structure and device design. (a) Optical image of rubrene–TCNQ charge-transfer interface device. The thicknesses of the isolated rubrene and TCNQ crystals are 1 μm and 13 μm, respectively. Scale bar, 100 μm. (b) Schematic ‘side view’ of a device structure, showing the electrical contacts, illuminated face and light direction in the photocurrent measurements. (c) Chemical structure of rubrene41and TCNQ (ref.42) molecules. (d) Different views of the crystal structure of rubrene (red) and TCNQ (yellow), according with the observation ‘side view’. These represent the views along the different axis direction (a,bandc), considering the crystal overlapping. Both structures present parallel stacks of molecules, with a herringbone configuration, typical of organic semiconductors. Figure 1: Rubrene–TCNQ molecular structure and device design. ( a ) Optical image of rubrene–TCNQ charge-transfer interface device. The thicknesses of the isolated rubrene and TCNQ crystals are 1 μm and 13 μm, respectively. Scale bar, 100 μm. ( b ) Schematic ‘side view’ of a device structure, showing the electrical contacts, illuminated face and light direction in the photocurrent measurements. ( c ) Chemical structure of rubrene [41] and TCNQ (ref. 42 ) molecules. ( d ) Different views of the crystal structure of rubrene (red) and TCNQ (yellow), according with the observation ‘side view’. These represent the views along the different axis direction ( a , b and c ), considering the crystal overlapping. Both structures present parallel stacks of molecules, with a herringbone configuration, typical of organic semiconductors. Full size image Single-crystal charge-transfer devices Rubrene–TCNQ crystalline charge-transfer interfaces were assembled manually, in air, by lamination of rubrene and TCNQ single crystals, a method frequently used in organic single-crystal field-effect transistors [14] . Such technique uses the ability of thin, usually 1 μm or thinner, and flat organic crystals to adhere to other even surfaces, metallic or insulators, by electrostatic forces and to other organic material layers, such as SAMs [25] or polymers (for example, polymethylmethacrylate [26] ). Examples arrive from different classes of molecular materials, such as the acenes [25] , [26] , [27] , [28] , metal phtalocyanines [29] , thiophenes [30] or the fulvalenes [31] . As long as the substrate roughness is smaller than just a few nanometres, thin organic crystals are flexible enough to adjust to most substrate surfaces. Even if the adhesion mechanism is not known in detail, it is commonly accepted that the surface bonding is based on electrostatic attraction, for instance by van der Waals forces, avoiding the crystal surface impairment by interdiffusion, layer mixing or chemical bonding. Such approach has lead, recently, to the discovery of a new interfacial two-dimensional electronic system by laminating different insulators, molecular crystals, TCNQ and tetrathiafulvalene (TTF) [21] . In the TTF–TCNQ system, charge transfer occurs at molecular scale in the interface of the two crystals, forming an electronic state with metallic characteristics, and in the absence of the Peierls transition, a typical transition of one-dimensional systems, such as the charge-transfer salt TTF–TCNQ (refs 32 , 33 ). Other approaches have also been used to induce higher conductivity at the surface of an organic crystal, such as through surface modification with SAMs, where surface conductivity was shown to depend on the electron-withdrawing ability of the top material [17] . These first examples of organic single-crystal heterojunction are representative of the possibility of new physical phenomena arising at the junction of organic crystal surfaces. With so many available molecular compounds, the combination of different donor and acceptor materials is vast, leading to different interfacial behaviour. This can be observed in recent examples of crystal on crystal lamination. Conjugating tetramethyltetraselenafulvalene and TCNQ crystals, for instance, forms a small-gap semiconductor system [34] , whereas in PDIF-CN 2 ( N,N′ -1 H ,1 H -perfluorobutyl dicyanoperylenecarboxydiimide) and rubrene system the valence band of the electron donor (rubrene) and the conduction band of the electron acceptor (PDIF-CN 2 ) are practically aligned [35] . As a result, the interfacial electron density presents a linear dependence of the temperature. This last example represents the first Schottky-gated organic heterostructure, demonstrating the potential of charge-transfer interfaces as a valuable tool to analyse organic–organic interfaces. Transport measurements The rubrene–TCNQ interface was found to have a resistance per square similar to the tetramethyltetraselenafulvalene–TCNQ system. In more than 30 samples assembled and measured in air, at room temperature, resistance values were lower than 20 MΩ, presenting a minimum value of 0.45 MΩ. A typical value of resistance per square of the interface is ~2 MΩ, which is more than three orders of magnitude smaller than the resistance of individual rubrene and TCNQ single crystals (>1 GΩ). In Fig. 2a , a typical I–V curve measured for the rubrene–TCNQ interface is shown. The mechanism associated with the observed higher current density at the interface is probably related to band bending due to the electrostatic potential created by polarization effects that ultimately lead to charge transfer from the HOMO of rubrene to the LUMO of TCNQ (ref. 34 ). In addition, the hybridization of the interfacial molecules of TCNQ–rubrene is likely to be quite small, comparable to the weak coupling between molecular planes observed in the individual constituents. This, most likely, leads to an interfacial conductivity constituted by two conductive layers with equal but opposite charge, one due to holes in the HOMO band of rubrene and the other due to electrons in the LUMO of TCNQ. 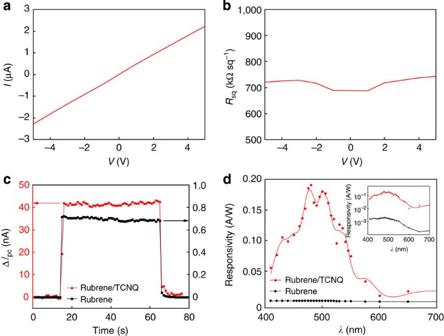Figure 2: Rubrene–TCNQ interface transport measurements and photoresponse. (a) I–V curve of a rubrene–TCNQ device. Measurements were performed in air, at ambient temperature and pressure. All measured samples exhibit a large electrical conductance, reaching five orders of magnitude higher than the individual TCNQ and rubrene crystals. (b) Normalized resistance of a rubrene–TCNQ sample. (c) Photocurrent response of rubrene–TCNQ interface (red) and rubrene crystals (black) at 500 nm illumination, taken at 5 V applied between the contacts. Rubrene–TCNQ response is ~2 orders of magnitude higher than rubrene’s response. (d) Spectral responsivity of rubrene (black) and rubrene–TCNQ (red). Such different response is quantified by differences in quantum efficiency of photocurrent generation. Figure 2: Rubrene–TCNQ interface transport measurements and photoresponse. ( a ) I–V curve of a rubrene–TCNQ device. Measurements were performed in air, at ambient temperature and pressure. All measured samples exhibit a large electrical conductance, reaching five orders of magnitude higher than the individual TCNQ and rubrene crystals. ( b ) Normalized resistance of a rubrene–TCNQ sample. ( c ) Photocurrent response of rubrene–TCNQ interface (red) and rubrene crystals (black) at 500 nm illumination, taken at 5 V applied between the contacts. Rubrene–TCNQ response is ~2 orders of magnitude higher than rubrene’s response. ( d ) Spectral responsivity of rubrene (black) and rubrene–TCNQ (red). Such different response is quantified by differences in quantum efficiency of photocurrent generation. Full size image The dispersion of resistance values measured in the interfaces (0.45–20 MΩ) is mainly related with different device quality, as well as the possibility of some conduction anisotropy originated by different orientation of the two crystals. It is well known that charge transport in organic semiconductors can differ along different crystal directions [36] . As the lamination process is manual, it becomes difficult to align both crystals always in the same direction. Moreover, all measurements were done with two-terminal contact configuration, including contact resistance, which is, in general, large [21] and has a higher impact on smaller samples. The fact that the sample length varied from 100 to 600 μm also leads to different relative contribution from contact resistance. Photophysics of the crystalline charge-transfer interface The absorption spectra of single crystals of the individual constituents rubrene and TCNQ, as well as the rubrene–TCNQ interface, are shown in Fig. 3a . No obvious change in absorption was observed when rubrene was laminated onto TCNQ in the studied spectral range, the interface spectrum being equal to the sum of the two spectra of the individual materials. Such observation, the lack of new absorption bands or a shift in the spectrum, indicates that the properties of the crystalline charge-transfer interfaces do not originate from new species created on the heterojunction due to chemical modifications, but rather from pure electronic interactions. 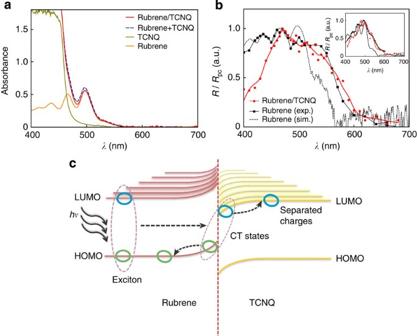Figure 3: Absorption spectra and photoresponse analysis. (a) Rubrene (orange), TCNQ (dark yellow) and rubrene–TCNQ interface (red) absorption spectra measured with unpolarized light at normal incidence with respect to the largest facet of the crystals. The absorbance of the isolated rubrene crystal (2.6 μm thick) was rescaled to match that of the crystal in the interface (1 μm thick). The interface absorption spectrum is equal to the sum of rubrene and TCNQ individual absorption spectra (blue) and no additional band is observed. Therefore, there are no evidences of formation of new chemical entities at the interftace. (b) Comparison between an experimental spectrum of rubrene (black squares), rubrene–TCNQ interface (red circles) and a simulated photoresponse spectrum for the isolated rubrene crystal (dashed line), obtained using eq. 1 in18withLEX=5 μm. In the main panel, TCNQ is laminated on top rubrene (both thickness ~7 μm), whereas the inset shows an interface with rubrene on top of TCNQ (rubrene 1 μm thick, TCNQ 13 μm), smoothed using a fourth-degree polynomial. In each graph, the thickness of rubrene is similar to the rubrene in the corresponding interface. The photocurrent spectra of the interfaces follows the photocurrent spectra of isolated rubrene of similar thickness. (c) Schematic representation of the interface energy diagram and photocurrent generation. Upon light exposure, an exciton is formed on rubrene. Following the exciton diffusion to the rubrene–TCNQ interface, the hole and electron are efficiently separated due to a charge-transfer process. This mechanism is assisted by an interfacial band bending. Figure 3: Absorption spectra and photoresponse analysis. ( a ) Rubrene (orange), TCNQ (dark yellow) and rubrene–TCNQ interface (red) absorption spectra measured with unpolarized light at normal incidence with respect to the largest facet of the crystals. The absorbance of the isolated rubrene crystal (2.6 μm thick) was rescaled to match that of the crystal in the interface (1 μm thick). The interface absorption spectrum is equal to the sum of rubrene and TCNQ individual absorption spectra (blue) and no additional band is observed. Therefore, there are no evidences of formation of new chemical entities at the interftace. ( b ) Comparison between an experimental spectrum of rubrene (black squares), rubrene–TCNQ interface (red circles) and a simulated photoresponse spectrum for the isolated rubrene crystal (dashed line), obtained using eq. 1 in [18] with L EX =5 μm. In the main panel, TCNQ is laminated on top rubrene (both thickness ~7 μm), whereas the inset shows an interface with rubrene on top of TCNQ (rubrene 1 μm thick, TCNQ 13 μm), smoothed using a fourth-degree polynomial. In each graph, the thickness of rubrene is similar to the rubrene in the corresponding interface. The photocurrent spectra of the interfaces follows the photocurrent spectra of isolated rubrene of similar thickness. ( c ) Schematic representation of the interface energy diagram and photocurrent generation. Upon light exposure, an exciton is formed on rubrene. Following the exciton diffusion to the rubrene–TCNQ interface, the hole and electron are efficiently separated due to a charge-transfer process. This mechanism is assisted by an interfacial band bending. Full size image The photoconductivity measurements were carried out on the largest facet ( a , b ) of the crystals (see Fig. 1b ), with coplanar contacts geometry, both for rubrene and rubrene–TCNQ interface. TCNQ photoresponse was also measured, but was found to be negligible at the studied wavelengths. This device geometry allows eliminating several problems arising in the usual sandwich layering metal/organic donor/organic acceptor/metal of thin-film measurements. Among the known constrictions are the quenching of excitons near the metal/organic interface, reflection losses of the metal film and metal interdiffusion onto the organic surface [37] , which lead to inaccurate results and poor device performance. In all experiments, it was always the top surface of the crystals that was illuminated, at normal incidence, whereas the photocurrent was measured in the b axis direction. Several experiments were executed to determine the effect of layering an acceptor crystal onto a donor crystal on the exciton dissociation. To account for contributions from the individual components, both rubrene and TCNQ crystals, as well as rubrene–TCNQ interfaces were analysed. As it was difficult to assemble the donor–acceptor interface in the same rubrene crystals used for photoconductivity measurements, different crystals were used. This approach also diminishes the possibility of rubrene surface degradation with time, exposed to light, air and dust. As can be seen in Fig. 2c , rubrene crystals present photoconductivity at 500 nm, with a photocurrent Δ I PC ≡ I illum − I dark ≈0.7 nA at an applied voltage of 5 V between contacts. However, in the same experimental conditions, the induced photocurrent in a rubrene–TCNQ interface with similar dimensions is orders of magnitude higher (Δ I PC ≡ I illum − I dark ≈42 nA in Fig. 2c ). At the same applied voltage, the TCNQ photoconductivity is negligible when compared with rubrene and with rubrene–TCNQ interface photoconductivity, consistent with previous observations [24] . In Fig. 3b , the photocurrent action spectra of rubrene–TCNQ interfaces are compared with the photoresponse of isolated rubrene crystals in the studied wavelength range (400–700 nm). The main panel of Fig. 3b shows the photocurrent spectra of an interface irradiated through the TCNQ surface, whereas the inset shows the spectrum of an interface irradiated through the rubrene surface. In all photocurrent spectra, the typical vibronic progression of rubrene can be observed [38] . However, the intensity modulation of the vibronic progression is particularly attenuated in the photocurrent action spectra with thicker rubrene crystals (main panel of Fig. 3b ), when compared with the absorption spectrum of rubrene. This can be explained by the thickness of rubrene, which determines the distribution of excitons inside the crystal, the fraction of absorbed photons at each wavelength and the probability of excitons generated at a certain depth to reach the interface. In fact, the photocurrent spectra is proportional to the integral of α . I 0 .exp(− α ( λ ) x ).exp(− x / L EX ) d x , where x is the direction perpendicular to the crystal surface and I 0 is the incident photon flux [18] . The observed attenuation, both in isolated rubrene crystals and the interfaces, is in accordance with simulated photocurrent spectra, using a typical exciton length of isolated rubrene crystal [23] , 5 μm, and the corresponding crystal thicknesses ( Fig. 3b ). This agreement constitutes an evidence of the participation of long-lived excitons, with diffusion lengths in the micrometre scale, in the generation of charge carriers. Such long-lived excitons have been previously identified in rubrene single crystals as triplet excitons generated via singlet fission [18] . The comparison of the simulated and experimental photoconductivity spectra evidences a systematic increased efficiency of the 534 nm band, both in the isolated rubrene crystals and interfaces. This transition at 534 nm corresponds to the HOMO–LUMO transition, for both ground and excited state in the vibrational ground state, and it is only allowed for light polarized along the c axis [38] . However, as shown in the absorption spectra, the observation of the band at 534 nm for unpolarized light at normal incidence with respect to the ( a , b ) plane is not uncommon, owing to small deviations from normal incidence and surface quality of the crystals [38] . The same light-polarization effects are also responsible for the observed enhanced photocurrent at 534 nm in the experimental spectra. In general, the photocurrent spectra of rubrene–TCNQ interfaces follow the spectra of the rubrene crystal of similar thickness. The only difference worth mentioning is the reduced photocurrent efficiency upon excitation at shorter wavelengths, below 450 nm (main panel in Fig. 3b ). When the 7-μm thick TCNQ crystal is on the top of the irradiated surface, it absorbs most of the light at 430 nm and only 0.02% of the incident photons reach the interface. This effect would lead to an almost complete suppression of the photoresponse at these wavelengths if rubrene excitons were the only ones generating current. The fact that the drop in the photocurrent efficiency is not proportional to the light reaching the interface indicates that excitons formed in TCNQ are also contributing to the photoconductivity. An apparently similar reduction effect is observed when rubrene is layered on top of TCNQ (inset in Fig. 3b ). However, this effect is fully understood on the basis of the reduced thickness of the crystal (1 μm) and the decay in the absorption coefficient at shorter wavelengths, and is supported by the agreement between the photoconductivity spectra of the interface and the isolated rubrene crystal. The nearly exact overlap of the photoconductvity spectra of isolated rubrene with that of the interfaces, without any significant shifts observed in the wavelength of the maximum intensity nor the observation of new bands in the interface spectrum, is an undeniable evidence that no new species formed at the interface are contributing to the electrical properties of the crystalline heterojunctions, as it could be initially anticipated from the absorption spectra. This observation matches well with the electronic description of an interfacial system with two separate conductive layers, holes in rubrene and electrons in TCNQ, weakly coupled, and in which rubrene has the most important contribution to exciton generation, as represented in Fig. 3c . To be able to compare results, the acquired data was normalized according to sample size, irradiation area and light intensity, into responsivity values, R=I pc /P exc , where I pc is the photocurrent intensity normalized by the irradiated area and P exc is the photon flux ( Fig. 2d ). All rubrene–TCNQ interface samples presented R ~3 orders of magnitude higher than single-crystal rubrene, with values reaching 1 A W −1 , whereas in rubrene the responsivity is at best ~1 × 10 −3 A W −1 . As R = ηq / hν ( η is the quantum efficiency, q is the elementary charge and hν is the photon energy), such low values of R on isolated rubrene are demonstrative of the small quantum efficiency of the photocurrent generation (0.5%). However, in rubrene–TCNQ interfaces the external quantum efficiency reaches 100% for samples presenting R ~0.4 A W −1 (~50% of all measured samples). The significant quantitative difference between a single-component device and a device combining a single crystal of a donor with a single crystal of an acceptor can be explained by a polarization effect on the interfacial rubrene and TCNQ molecules, due to electron affinity differences, which induces a dipolar layer at the interface. An interpretative diagram is represented in Fig. 3c . In this description, the optical excitons originally generated in the bulk of rubrene can diffuse to the interface where they dissociate into free charges by electron transfer from the LUMO of the electron donor rubrene to the LUMO of the electron acceptor TCNQ. The charge carriers will then diffuse along different sides of the interface. The interfacial band bending increases the offset between the LUMO of rubrene and the LUMO of TCNQ, affecting the excess energy of the bound electron in TCNQ and, eventually, leading to a higher efficiency of generation of free electrons. A fraction of the samples of rubrene–TCNQ charge-transfer interface (~25%) presented responsivity values corresponding to quantum efficiencies higher than 100%, with 1< R <5 A W −1 . Even if all the singlet excitons formed upon excitation would lead to charge carriers via a singlet fission mechanism, the responsivity would be, at best, 0.8 A W −1 , due to a charge-carrier generation efficiency of η =2. Thus, singlet fission alone cannot be responsible for the high responsivity values. A reasonable explanation to this effect is a small internal gain mechanism due to differences in the carrier mobility. This would generate differences in the transit time, τ , of the hole and the electron, leading to a larger gain factor [39] (see Fig. 1b for illustration of the effect). The results here presented constitute the first photoresponse characterization of single-crystal charge-transfer interfaces. The increase of responsivity of the rubrene–TCNQ single-crystal heterojunction shows that it is possible to modify the interfacial energy with a tremendous increase in the photoexciton dissociation. It is expectable that the combination of the donor and acceptor crystals leads to an interfacial band bending, thus lowering the necessary energy for charge separation and favouring the exciton dissociation. This would be the main role of the charge-transfer interface, as well as to separate the generated carriers into the two conductive layers, with holes carried by the HOMO band of rubrene and electrons carried by the LUMO band of TCNQ. These two effects, improvement of charge generation and separation, contribute significantly to the unambiguous increase of quantum efficiency. The ability of the crystalline heterojunctions to combine high quantum efficiency with the high mobility observed in single crystals, and at low bias, is unique in organic devices. This observation may open a new direction to unprecedented photocurrent efficiencies in organic photovoltaic diodes. Interface fabrication Rubrene and TCNQ single crystals were grown by optimized physical vapour transport, using argon as a carrier gas, a common method used on organic materials [40] . Both rubrene and TCNQ powder (Sigma-Aldrich) were sublimated at ~300 °C and 270 °C, respectively. Rubrene–TCNQ interfaces were assembled by lamination (see [22] for more details), in different substrates (polydimethylsiloxane or glass) according to crystal thickness and measurement specifications. The contacting surface was the ( a , b ) plane both for rubrene and TCNQ (see Fig. 1 ). Bottom-layer crystals used in glass were less than 2 μm thick to ensure adhesion to substrate, whereas on adhesive polydimethylsiloxane a thicker bottom-layer crystal could be used (0.2–30 μm). Colloidal graphite paint was deposited on the conductive interface, always after crystal lamination, usually at the edge of the two crystals, and was used as electrical contacts. Contact distance separation depended on the interface size, differing from 100 up to 1,500 μm. Characterization measurements All measurements were done in air, and samples could resist for months without particular storing care, showing no sign of degradation. The crystal thickness was determined using a Dektak 3030ST profilometer. Electrical measurements were done using a Keithley 237 source-measure unit. In photoconductivity measurements, the top crystal surface, corresponding to the ( a , b ) plane, was irradiated at normal incidence using an unpolarized monochromatic light in the 400–700 nm range, obtained by coupling the light from a 250-W quartz tungsten halogen lamp into a double monochromator set-up. A long-pass filter with a 550 nm cut-on wavelength was used to avoid interference from second-order diffraction. A calibrated Si photodiode (Thorlabs, S121C) was used to measure the incident power. Absorption spectra were collected using an Ocean Optics QE65Pro spectrometer with unpolarized light from a deuterium tungsten halogen light source (ScanSource ABS, 200–1100, nm) at normal incidence with respect to the largest natural facet of the crystals, ( a , b ). How to cite this article: Alves, H. et al. Photoconductive response in organic charge transfer interfaces with high quantum efficiency. Nat. Commun. 4:1842 doi: 10.1038/ncomms2890 (2013).